Enhanced role of eddies in the Arctic marine biological pump The future conditions of Arctic sea ice and marine ecosystems are of interest not only to climate scientists, but also to economic and governmental bodies. However, the lack of widespread, year-long biogeochemical observations remains an obstacle to understanding the complicated variability of the Arctic marine biological pump. Here we show an early winter maximum of sinking biogenic flux in the western Arctic Ocean and illustrate the importance of shelf-break eddies to biological pumping from wide shelves to adjacent deep basins using a combination of year-long mooring observations and three-dimensional numerical modelling. The sinking flux trapped in the present study included considerable fresh organic material with soft tissues and was an order of magnitude larger than previous estimates. We predict that further reductions in sea ice will promote the entry of Pacific-origin biological species into the Arctic basin and accelerate biogeochemical cycles connecting the Arctic and subarctic oceans. Evaluating the responses of biogeochemical cycles to decreasing sea ice is important to predict long-term trends in fishery resources [1] . Improved summer light conditions have been reported to enhance planktonic photosynthesis in the Eurasian pelagic area of the Arctic Ocean [2] , [3] , [4] . Furthermore, the accumulation of nutrient-poor freshwater suppressed the primary production of phytoplankton in the central Canada Basin during the 2000s (ref. 5 ). Biological pumping of particulate organic carbon (POC), which is one of the sequestration mechanisms of atmospheric CO 2 to the deep sea, has been reported to be ineffective in the cryopelagic Canadian Arctic deep basins [6] . Whereas primary productivity of phytoplankton could be modest even under sea ice cover; low abundance of ballast particles such as shell-bearing micro-planktons might have prevented biological materials from sinking towards deep layers [6] . In contrast, lateral transport of resuspended bottom sediments played a role in oceanic carbon sink in the western Arctic off-shelf regions [7] . These findings were obtained by time series sediment trap measurements in the deep Canada Basin [6] , the Canadian Beaufort shelves [8] , [9] , [10] , [11] , [12] , the northern Laptev Sea [2] and the Nordic seas [13] ( Fig. 1 ). However, there are many gaps to fill to achieve a comprehensive explanation of the spatial and temporal variability of biological pump processes under rapid environmental changes of the Arctic Ocean. The relative contribution of the lateral transport of shelf-origin materials to basin interiors remains uncertain. The western Canada Basin and the Chukchi Borderland, which have experienced a remarkable reduction of sea ice and substantial biological shifts during the early 21st century, are located downstream of Pacific-origin water that obtains heat, nutrients and organic material over the shallower Chukchi shelf. Thus, further investigations of the physical and biogeochemical properties along the Pacific water pathway will provide valuable information regarding communication between the Bering Sea and the central Arctic. 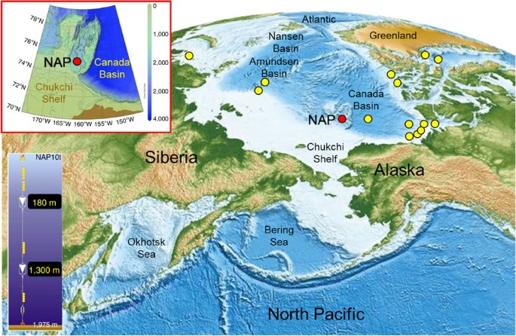Figure 1: Topography map in the Arctic-subarctic regions. Red dots show the location of Station NAP, where our sediment trap (bottom left inset) has been deployed since October 2010. Yellow dots show the locations of previous year-long bottom-tethered sediment traps (See alsoFig. 1in a Honjo’s work6). Topography was figured based on NGDC-ETOPO1 data50. Figure 1: Topography map in the Arctic-subarctic regions. Red dots show the location of Station NAP, where our sediment trap (bottom left inset) has been deployed since October 2010. Yellow dots show the locations of previous year-long bottom-tethered sediment traps (See also Fig. 1 in a Honjo’s work [6] ). Topography was figured based on NGDC-ETOPO1 data [50] . Full size image We detect a significant amount of sinking biogenic materials with particulate organic nitrogen (PON) using measurements from sediment traps deployed in the Northwind Abyssal Plain (NAP; Fig. 1 ) since autumn 2010 ( Supplementary Fig. 1 ). We then address the background mechanisms and possible future conditions of the biological pump from the viewpoint of shelf water transport using an eddy-resolving (5-km grid size) framework in a pan-Arctic sea ice-ocean model. Our findings reveal the effective role of Beaufort shelf-break eddies in biological pumping from the Chukchi shelf to the Canada Basin. Because these eddies are generated in summer immediately after shelf blooms of phytoplankton, biological activity can continue even during eddy migration towards the central Arctic. Whereas the so-called ‘lateral biological pump’ have meant the resuspension and eddy-induced transport of bottom sediments composed of old carbon, the presented process may sustain marine ecosystems in seasonal ice zones of the Arctic basins. Seasonality of biogenic particle fluxes at Station NAP In response to recent marked reduction in the western Arctic sea ice [14] , the unique seasonality of lower-trophic marine ecosystems and the significant contribution of lateral transport to fresh particle fluxes were observed using sediment trap measurements at Station NAP. In the Chukchi Borderland, polar night and sea ice freezing begin in mid-October ( Fig. 2a,b ). The total mass flux (TMF) and biogenic particle fluxes had their peaks in November–December of 2010 and 2011, in addition to July–August 2011 ( Fig. 2c ). The trapped particles mainly consisted of lithogenic silty-clay materials, as previously observed for spring seasons using the ice-tethered drifting sediment trap S97-120 m over the Chukchi Rise and the bottom-moored trap at Station CD04-3,067 m in the cryopelagic Canada Basin [6] . However, the other contents remarkably differed among these surveys. The diatom frustules and/or valves, and micro-zooplankton with soft tissues were commonly observed in both shallow and deep trap samples at Station NAP, whereas the organic material captured by the preceding traps in the deep Canada Basin consisted of old carbon with average age of ~\n1,900 years [15] . The relative abundance of biogenic particles increased during the high TMF periods at Station NAP ( Fig. 2c ). In late November 2011, the trapped fluxes of POC and PON were 124.5 μmol-C m −2 per day and 12.6 μmol-N m −2 per day, respectively ( Supplementary Data ). The C/N ratio of ~\n10 suggested a mixture of autochthonous microplankton and terrigenous/old organic materials. In the decomposition of organic materials, nitrogen is respired faster than organic carbon [16] . On the basis of this relationship, the concentration of marine POC was estimated from the total carbon content and POC/N molar ratios of marine plankton (C/N=5–7) [16] and the mass balanced mean (C/N=37.1) [17] of terrigenous organic materials, which consisted of colloidal organic carbon, low molecular weight dissolved organic carbon, and POC transported from the Yukon River [18] . According to this method, marine origin organic carbon was estimated to account for more than 84.3% of the total organic carbon ( Supplementary Fig. 2 ). This ratio and the substantial amount of micro-zooplankton with soft tissues implied that a great part of POC collected at Station NAP was fresh. These characteristics were markedly different from previous observations in the western Arctic basin. Approximately 40% of the annual flux of organic material (except organic material such as the gelatinous houses of zooplankton Appendicularians in the >1 mm size fraction) was observed during November–December. The biogenic opal flux, which was mainly composed of diatom frustules and/or valves, was the greatest in late November 2010 rather than in summer ( Fig. 2c ). 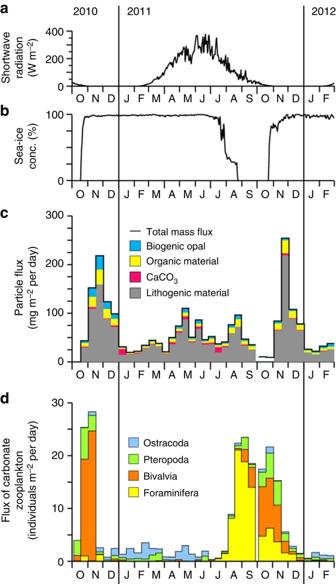Figure 2: Shortwave radiation, sea ice concentration and particle fluxes at Station NAP. Time series from 4 October 2010 through 1 March 2012. (a) Downward shortwave radiation at the surface of sea ice and ocean (after sea ice opening) from NCEP-CFSR (W m−2). (b) Sea ice concentration from NCEP-CFSR (%). (c) Cumulative bulk component and total mass flux of 36 trapped particle samples (mg m−2per day]. Replicate analysis was not conducted because of limited sample volume. The blank in bulk component represents no data. The water depth of the shallow trap was ~\n180 m during the first deployment through 27 September 2011, and approximately 260 m during the second deployment. (d) Fluxes of carbonate shell bearing micro-zooplankton (individuals m−2per day). Figure 2: Shortwave radiation, sea ice concentration and particle fluxes at Station NAP. Time series from 4 October 2010 through 1 March 2012. ( a ) Downward shortwave radiation at the surface of sea ice and ocean (after sea ice opening) from NCEP-CFSR (W m −2 ). ( b ) Sea ice concentration from NCEP-CFSR (%). ( c ) Cumulative bulk component and total mass flux of 36 trapped particle samples (mg m −2 per day]. Replicate analysis was not conducted because of limited sample volume. The blank in bulk component represents no data. The water depth of the shallow trap was ~\n180 m during the first deployment through 27 September 2011, and approximately 260 m during the second deployment. ( d ) Fluxes of carbonate shell bearing micro-zooplankton (individuals m −2 per day). Full size image Whereas a summer maximum flux of sinking biogenic materials is usually explained by phytoplankton bloom around Station NAP, the high fluxes in early winter are not interpreted as merely reflecting the seasonal cycles of local biological productivity. Photosynthesis activity is not likely to occur under the low light conditions created by sea ice cover and polar night after mid-October ( Fig. 2a,b ). The high winter flux of sinking micro-zooplankton must be derived primarily from allochthonous materials, including clay-silt-sized minerals. Another clue for the shelf-to-basin material advection included the seasonal dominance of planktic juveniles of coastal bivalvia in the calcareous micro-zooplankton during the high TMF periods from late autumn to early winter ( Fig. 2d ). Bivalve larvae were most dominant from the Bering Strait to the eastern Chukchi shelf, whereas their occurrence was rare in the basin interior (Kimoto, unpublished data). Most calcareous micro-zooplankton specimens in the analysed samples contained soft tissues, and thus were likely alive until the periods shortly before being trapped. Our trap data suggested that the particle fluxes of biogenic and lithogenic materials (LMs) around the Northwind Abyssal Plain were more massive than the previous records in the western Arctic basin [6] . A major part of this contrast can be explained by the pathway and transport mechanism of shelf-origin water. It was suggested that a distinct warm eddy propagating north of the Chukchi shelf break provided a substantial amount of shelf-origin heat and nutrients to the Canada Basin interior [19] , [20] . Because our sediment traps were located 70–100 km away from the Chukchi shelf break, the development and migration of such eddies would be a key phenomenon in the lateral transport of fresh organic materials and in explaining the early winter increase in sinking particle fluxes at Station NAP. Roles of shelf-break eddies in biological pump A seasonal experiment using our pan-Arctic sea ice ocean model demonstrated that the PON flux at Station NAP initially increased in July and reached summer and early winter peaks at depths of 180 and 1,300 m ( Fig. 3 ). At the shallower depth, the first peak reached 52 μmol-N m −2 per day on 18 September, and the early winter peak reached 55 μmol-N m −2 per day on 5 November. These modelled fluxes were larger than those derived from our shallow sediment trap data, but the modelled flux values at the greater depth were similar to the corresponding trap data. Assuming 1 mmol-N~\n80 mgC (Redfield ratio), the carbon sink derived from the simulated PON flux at a 180 m (1,300 m) depth was 258 (59) mgC m −2 from May to December. In this respect, our model closely reproduced the seasonal transitions in sea ice concentration and plankton productivity at Station NAP ( Supplementary Fig. 3 ). The sea ice concentration in the COCO model rapidly decreased to zero in mid-August. The modelled timing of ice decline was ~\n2 weeks later than that shown by the satellite product, whereas the freezing period beginning in October was nearly identical between our model and the satellite data. The downward shortwave radiation from National Centers for Environmental Prediction-Climate Forecast System Reanalysis (NCEP-CFSR) peaked at 339 W m −2 on 21 May 2010, and the shortwave radiation absorbed at the ocean surface varied depending on sea ice concentration, reaching a maximum of 122 W m −2 on 17 August. In general, light limitation impedes photosynthesis activity of phytoplankton during the ice cover period. However, it was suggested that the formation of melt ponds played an essential role in the under-ice massive phytoplankton bloom [21] . In addition, the simulated primary production began in June, before sea ice disappearance, and continued until early October in our model, which did not include light penetration through the sea ice column yet. Therefore, we infer that shortwave radiation into the open water fraction in sea ice cracks also contributes to under-ice blooms. The total primary production during the model integration period reached 344 mmol-N m −2 (~\n28 gC m −2 ). The ship-based measurements revealed an annual primary production of 20 gC m −2 per year with a summertime peak of 0.32 gC m −2 per day at the edge of the Canada Basin [22] . Several model simulations have supported these values for the western Arctic shelf-basin boundary region [23] , [24] , [25] , [26] . The ratio of zooplankton grazing to total primary production was 39% in our model, within previous estimates from 20 to 50% (refs 27 , 28 ). Thus, the primary and secondary productions at Station NAP in our model were consistent with many other studies. 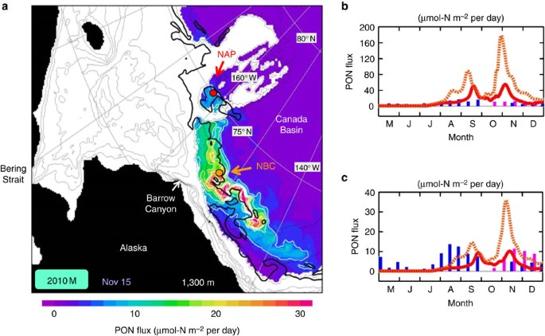Figure 3: Modelled PON flux. (a) PON flux at a depth of 1,300 m on 15 November in the 2010 M case (μmol-N m−2per day). The modelled tracer concentration of shelf bottom water at 150 m depth is 0.1 along black contours. Thin grey contours show sea bottom bathymetry. (b,c) The flux time series at (b) 180 and (c) 1,300 m depths; pink and blue bars represent the observed fluxes in 2010 and 2011, respectively. The modelled fluxes in the 2010 M case at Station NAP and north of Barrow Canyon (NBC) are shown by solid red and dashed orange lines, respectively. Figure 3: Modelled PON flux. ( a ) PON flux at a depth of 1,300 m on 15 November in the 2010 M case (μmol-N m −2 per day). The modelled tracer concentration of shelf bottom water at 150 m depth is 0.1 along black contours. Thin grey contours show sea bottom bathymetry. ( b , c ) The flux time series at ( b ) 180 and ( c ) 1,300 m depths; pink and blue bars represent the observed fluxes in 2010 and 2011, respectively. The modelled fluxes in the 2010 M case at Station NAP and north of Barrow Canyon (NBC) are shown by solid red and dashed orange lines, respectively. Full size image Because shelf bottom water is considered to be the crucial nutrient source for biological production in the basin area [29] , its pathway was addressed using a coloured passive tracer in the model experiment ( Supplementary Fig. 4 ). In the seasonal experiment, the COCO model reproduced three branches of northward current in the Chukchi shelf. The western path followed Herald Canyon, the middle path followed the Central Channel and the eastern branch followed the Alaskan coast. Part of the current passing through each branch eventually converged towards Barrow Canyon, creating the strong canyon jet. The anti-cyclonic Beaufort Gyre circulated in the Canada Basin. The simulated concentration of the shelf bottom water tracer showed that the bottom water was well mixed below the seasonal stratification formed by summer sea ice melting and solar heat input north of the Bering Strait and along the pathway of major shelf circulation. In addition, part of the shelf bottom water was transported into the southern Canada Basin by the Beaufort shelf-break eddies. The tracer was distributed at a depth of ~\n20–180 m within each eddy. The tracer signal clearly indicated that the shelf bottom water reached Station NAP at the peak timing of PON flux in this case ( Fig. 3 ). Moreover, a distinct minimum-temperature layer, which was isolated from the surface mixed layer, appeared at a depth of 100–200 m from October to December. This cooling event was detected by the sediment trap sensors ( Supplementary Fig. 1 ) and indicated the lateral advection of cold water mass. Wind-driven Ekman transport is also a player for shelf-basin exchange in the surface layer. However, shelf bottom water was not directly transported towards the basin interior across the sharp shelf break in the present experiment. Thus, surface Ekman transport would not explain the early winter peak of sinking mass flux at Station NAP. Here, we propose that mesoscale eddies originating in the vicinity of the Barrow Canyon mouth and the Beaufort shelf break play an important role in biological pumping in the western Arctic basin. Our model reproduced both cold and warm shelf-break eddies [30] ; ( Fig. 4 ). The detailed generation mechanism of shelf-break eddies was described in Supplementary Note . The hydrographic and biogeochemical properties of eddies reflected the environment of Barrow Canyon during their generation ( Supplementary Fig. 5 ). The vertical profiles of physical and ecological variables at the centres of cold and warm eddies were tracked across the eddy life stages ( Fig. 5 ; Supplementary Fig. 6 ). Although the core temperatures of each eddy were altered by mixing with surrounding basin water, as shown by the tracer concentration of shelf bottom water, the cold and warm cores persisted at least until December. One such cold eddy migrated westward along the pathway of basin-wide Beaufort Gyre circulation and passed Station NAP in November ( Fig. 4 ). This eddy, generated in June, carried near-freezing shelf water ( Fig. 5a ). The cold eddy captured an initial surface bloom of phytoplankton from June. According to enhanced light penetration into the water column and surface nutrient depletion, the peak of phytoplankton biomass shifted to a subsurface layer in July and August, and then gradually disappeared after September. Zooplankton grazing followed the phytoplankton bloom. A significant amount of zooplankton biomass remained even in November. Because of these phytoplankton bloom and zooplankton grazing, the PON concentration within the cold eddy increased from June to August in most of the water column and exceeded 10 μmol-N m −3 until the eddy passed Station NAP in November ( Fig. 5b ). Because the PON concentration within the cold eddy was higher than that in the surrounding basin water, the second peak of PON flux occurred in early winter at Station NAP. 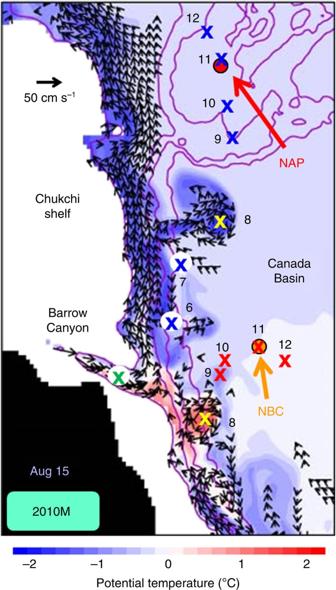Figure 4: Pathway of shelf-break eddies. Potential temperature (°C) (colour bar) and ocean horizontal velocity at a 100 m depth on August 15 in the 2010 M case. The unit vector is 50 cm s−1and vectors of velocity less than 5 cm s−1are hidden. Blue (red) crosses indicate the locations of cold (warm) eddy centres in each month (for example, ‘6’ denotes 15 June, ‘7’ denotes 15 July and so on). Yellow crosses are those on August 15, which is the same date as temperature and velocity plots. A green cross in the Barrow Canyon is referred inSupplementary Fig. 5. Purple contours show water depths of 100, 500, 1,000 and 2,000 m. Figure 4: Pathway of shelf-break eddies. Potential temperature (°C) (colour bar) and ocean horizontal velocity at a 100 m depth on August 15 in the 2010 M case. The unit vector is 50 cm s −1 and vectors of velocity less than 5 cm s −1 are hidden. Blue (red) crosses indicate the locations of cold (warm) eddy centres in each month (for example, ‘6’ denotes 15 June, ‘7’ denotes 15 July and so on). Yellow crosses are those on August 15, which is the same date as temperature and velocity plots. A green cross in the Barrow Canyon is referred in Supplementary Fig. 5 . 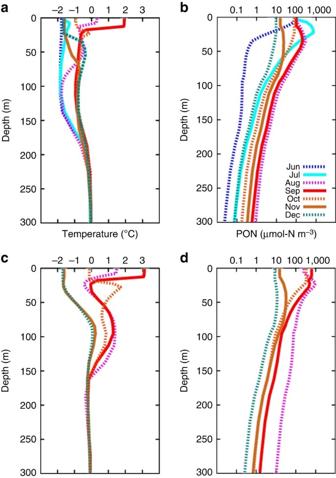Figure 5: Vertical eddy profiles. Vertical profiles of (a,c) potential temperature (°C) and (b,d) PON concentration (μmol-N m−3) at the centres of (a,b) cold and (c,d) warm eddies, whose locations are shown inFig. 4. See alsoSupplementary Fig. 6for other eddy properties. Purple contours show water depths of 100, 500, 1,000 and 2,000 m. Full size image Figure 5: Vertical eddy profiles. Vertical profiles of ( a , c ) potential temperature (°C) and ( b , d ) PON concentration (μmol-N m −3 ) at the centres of ( a , b ) cold and ( c , d ) warm eddies, whose locations are shown in Fig. 4 . See also Supplementary Fig. 6 for other eddy properties. Full size image As well as the cold eddies, warm eddies generated after the surface bloom over the shelf region had a subsurface peak of phytoplankton biomass in August. It was suggested that the time lag between the phytoplankton bloom following summer sea ice retreat in the Chukchi shelf and the generation of shelf-break eddies is an important index of biological regimes in the Canada Basin [31] . In our model experiment, the vertically integrated zooplankton biomass within the warm eddies were larger than those within the cold eddies. Warmer condition favours a series of export production. A distinct warm eddy with high chlorophyll and low nitrate concentration was observed by the R/V Mirai cruise during the later summer of 2010 (ref. 19 ). In contrast, the simulated warm eddy had a nitrate peak at the 50 m depth because its rotational flow took additional nutrient from surrounding water and because nitrogen recycling with decomposition of dissolved organic nitrogen (DON) and PON and nitrification from ammonium worked on nitrate recovery. Warm eddies generated after sea ice retreat in late summer had greater contribution to PON flux compared with cold eddies produced under sea ice in early summer. In the case of warm eddies, the PON concentration exceeded 100 μmol-N m −3 from the eddy generation period in August. The higher water temperatures in the ocean surface layer of warm eddies kept their pathways away from the sea ice cover; thus, both the warmer conditions and the greater light intensity favoured phytoplankton photosynthesis and subsequent zooplankton grazing. A higher PON flux was then localized in part of the southern Canada Basin ( Fig. 3 ), where baroclinic eddies traced. We checked the PON flux north of Barrow Canyon (NBC), where a warm eddy passed on 15 November ( Figs 3 and 4 ). The peak fluxes of 178 and 36 μmol-N m −2 per day at 180 and 1,300 m, respectively, were several times larger than those within the cold eddy at Station NAP. In the Mackenzie shelf region, it has been reported that the resuspension of shelf bottom sediments and cross-shelf transport of POC were induced by buoyancy-driven convection following winter sea ice formation [8] and by baroclinic eddies [7] , [11] . In contrast, our results showed that high plankton activity was accompanied by the development and migration of summer eddies in the downstream region of the Pacific water pathway. This eddy-induced biological pump would be enhanced by sea ice retreat. To address the impact of sea ice reduction on the early winter PON flux, we performed two additional experiments in which the sea ice thickness given as the initial condition on March 1 was multiplied by 2.0 or 0.5 in the entire model domain (named as Ice2.0 and Ice0.5 cases, respectively). The total sea ice extent on 1 October was 6.9 (3.9) × 10 6 km 2 in the Ice2.0 (Ice0.5) cases ( Fig. 6 ). The average summer sea ice extent during the 1990s was similar to the Ice2.0 case, and the 2012 sea ice margin was located farther north than that seen in the Ice0.5 case. The November mean PON flux was averaged in the southwestern Canada Basin, which was defined as being enclosed by 140°W, 160°W, 75°N and a 3,000 m isobath. The simulated flux below 200 m was 16 μmol-N m −2 per day in the Ice2.0 case, whereas it reached 32 μmol-N m −2 perday in the Ice0.5 case. These modelling results indicate that the magnitude of the biological pump might have doubled over the last two decades in the southwestern Canada Basin. This trend arose because the eddy-driven transport of shelf-origin nutrients and biological materials towards the Canada Basin was promoted. The modelled eddy properties in each case were summarized in Table 1 . The ‘Integrated PON of Eddy Grids (IPEG)’ was larger (smaller) in the Ice0.5 (Ice2.0) case than those in the 2010 M case in the southwestern Canada Basin. The factor for this difference could be attributed to changes in shelf bloom and eddy activity, respectively. The improved light conditions owing to sea ice reduction increased phytoplankton biomass in early summer. For example, the PON concentration per eddy volume, which was defined as ‘Averaged PON of Eddy Grids (APEG)’, increased from 88 μmol-N m −3 in the Ice 2.0 case to 139 μmol-N m −3 in the Ice 0.5 case on the seasonal average of June, July and August. The earlier shelf bloom hastened nutrient depletion and rapidly reduced the PON content per each eddy from summer to autumn. The APEG became the smallest in the Ice0.5 case during September, October and November. In contrast, the removal of sea ice drag increased the Barrow Canyon outflow and eddy kinetic energy [32] . The larger ‘Integrated Volume of Eddy Grids (IVEG)’ reflected the stronger eddy activity occurring under conditions of less sea ice. In addition, the enhanced eddy generation and development promoted greater PON export to the deep basin under less sea ice condition. We can indicate that eddy-induced lateral nutrient supplies to the euphotic zone have favoured the increasing phytoplankton growth in the Canada Basin, whereas the deepening nutricline in part caused by sea ice reduction may suppress primary productivity [5] , [19] . Thus, the environmental transition for lower trophic ecosystems in the marginal Beaufort Gyre, including the NAP area, differs from the situation in the central gyre. In addition, the recent acceleration of Beaufort Gyre was reported by drifting buoy measurements [33] . The faster gyre circulation is expected to reinforce the westward transport of Chukchi shelf water and to induce earlier peaks of PON flux at Station NAP. Now, we need to consider how far the area of high biological activity will spread in the near future and how ocean dynamics will contribute to the pan-Arctic marine ecosystem. Because mesoscale eddies have been detected in multiple shelf-basin boundary regions of the Arctic Ocean [34] , [35] , [36] , the ecological function of laterally transported organic materials is likely to gain more importance as a food source for plankton and higher-trophic organisms in the basin interior. 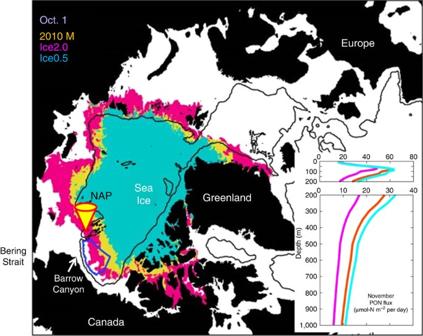Figure 6: Impact of sea ice reduction. Sea ice distribution on 1 October in the (orange) 2010 M, (pink) Ice2.0, and (sky blue) Ice0.5 cases. Black contours represent 1,000 m isobaths. The location of Station NAP is shown by a yellow cone. The inset shows the vertical profile of November mean PON flux in each case (μmol-N m−2per day). The average region is the southwestern Canada Basin, which is outlined by a blue contour. Figure 6: Impact of sea ice reduction. Sea ice distribution on 1 October in the (orange) 2010 M, (pink) Ice2.0, and (sky blue) Ice0.5 cases. Black contours represent 1,000 m isobaths. The location of Station NAP is shown by a yellow cone. The inset shows the vertical profile of November mean PON flux in each case (μmol-N m −2 per day). The average region is the southwestern Canada Basin, which is outlined by a blue contour. Full size image Table 1 Modelled eddy properties. Full size table Sediment trap measurements The bottom-tethered moorings with time series sediment traps (SMD26S-6000, NiGK Cooperation) have been deployed at Station NAP (75°N, 162°W, 1,975 m water depth) from 4 October 2010 to the present. The deployed sediment traps can collect 26 samples in one deployment. The initial deployment and turnaround of the sediment trap moorings were conducted by R/V Mirai and the Canadian Coast Guard Ship Sir Wilfrid Laurier. In the first year of deployment, sinking particle sampling was conducted by two time series sediment traps deployed at depths of 181–218 m (median; 184 m) and 1,318–1,339 m (median; 1,323 m) from 4 October 2010 through 27 September 2011. The open and close time for each sampling was 0:00. In the second year of deployment, two sediment traps were deployed at depths of 247–269 m (median; 258 m) and 1,357–1,367 m (median; 1,360 m) during the studied period from 4 October 2011 throughout 1 March 2011. In general, the trapping efficiency of sinking particles in sediment trap measurements is reduced by strong ocean circulation in the upper water column (above 1,000 m) [37] . We have already confirmed the insignificant impact of horizontal ocean currents on trapping efficiency at Station NAP [38] . In addition, the data logs of the pressure sensor attached to the shallower sediment trap showed that the moored trap depth was essentially constant during the sampling period ( Supplementary Fig. 1 ). Moreover, the TMF level at the shallow trap was not significantly lower than the one of the deep trap moored at 1,300–1,360 m. Therefore, the underestimation bias in sinking fluxes owing to trapping efficiency of the shallow trap was considered to be small. Analyses of trapped particles To preserve the trapped particles, each sample bottle was filled with pre-filtered deep sea water with 4% pH neutralized formalin before the sediment trap deployment. The collected sinking particle samples were sieved (1 mm mesh) to remove large swimmers, and the fine particle fraction (less than 1 mm) was equally split into appropriate aliquots for each analysis (1/10 to 1/1,000) using a rotary splitter Wet Sample Divider (WSD-10) of McLane Research Laboratories. For TMF analysis, 1/10 samples were filtered on polycarbonate filters (i.d. 47 mm, 0.4 μm pore size) and desalted with Milli-Q water. The filters were dried in a desiccator with diphosphorus pentoxide for a few days, and the dried filters were then weighed to obtain the total mass (TM). After weighting, the dried particles (5–10 dry mg) were used for analyses of POC, particulate inorganic carbon and nitrogen with a CHN Analyzer NCS2500, Thermo Quest. For POC analyses, the samples were decalcified in concentrated hydrochloric acid vapour. The PIC content was estimated as the difference between the total particulate carbon and POC contents. The concentrations of Si, Al, Fe, Ti, Mg and Ca (in approximately 20 mg samples) were analysed using ICP-AES. The LM concentration was estimated by using two methods: and Because the samples contained abundant clay minerals, the latter equation (2) using the mean crustal composition often showed inadequate value of the LM concentration. This error was most likely due to regional differences in the elemental composition of LM. Here, the equation (1) was used to calculate the LM concentration. To analyse the sinking assemblage of calcareous micro-zooplankton, 1/10 samples were used. All calcareous microzooplankton (foraminiferans, juvenile bivalvia, pteropods and ostracods) were picked out under an objective microscope. To analyse the diatom flora, 1/1,000 samples were used, and the analytical procedure followed our previous study [39] . Marine ecosystem model The pan-Arctic sea ice-ocean model comprised a physical ocean general circulation model, ‘Center for Climate System Research Ocean Component Model (COCO) [40] ’ version 4.9, and a lower trophic marine ecosystem model, ‘North Pacific Ecosystem Model for Understanding Regional Oceanography (NEMURO) [41] ’. We analysed the results of a seasonal experiment from March to December 2010 using an eddy-resolving version with a 5-km grid size (called as the 2010 M case). The initial sea ice and ocean physical fields were obtained from a decadal experiment from 1979 to 2012 using a 25-km grid version (updated from our previous experiments [42] , [43] ). In both experiments, the atmospheric forcing components were constructed from the NCEP-CFSR six-hourly data set [44] . The NEMURO model, which was originally developed to assess marine biology in the North Pacific, treats the concentrations of 11 biogeochemical variables on nitrogen and silicon cycles [41] . It has recently been confirmed to perform well across the global domain [45] , [46] and for pelagic primary productivity in the Arctic basins [47] , whereas the lack of sea ice ecosystem (for example, ice algal production) might have caused the summertime lag of PON flux in our experiment. Monthly climatological data of nitrate and silicate concentrations derived from the World Ocean Atlas 2009 (WOA09) [48] were used for restoring along the lateral boundary region of the model domain, and the March values were assigned to the initial fields. In our experiments, most parameter values such as the phytoplankton photosynthetic rate and the zooplankton grazing rate followed a precedent [47] . PON was generated from mortality and egestion processes of each plankton component. The decomposition rates from PON to ammonium and dissolved organic nitrogen were set to 0.1 per day at 0 °C, respectively. Increasing water temperatures enhanced these rates according to a traditional Q 10 relationship [41] . The sinking velocity of PON was prescribed from 2 m per day in the uppermost model layer to 200 m per day at 1,000 m depth following a cosine curve because the sinking of particulate organic materials generally accelerates with depths due to particle densification processes (for example, aggregation in shallow depths and elimination of light/fragile organic materials in middle depths) [49] . Below 1,000 m depth, the sinking velocity was maintained at 200 m per day. The modelled diatom species (PL in the NEMURO model) has somewhat larger biomass than other phytoplankton group (PS) in both the cold and warm eddies (not shown). Actually, there remain many uncertainties on nutrient profiles and dominant plankton species inside the shelf-break eddies. More information on eddy properties would help model formulation of advanced schemes such as variable sinking velocity of PON depending on plankton types. Geochemical fluxes from sea bottom sediments were considered crucial nutrient sources not only in the Chukchi shelf but also in the basin area, because the spread of ammonium-rich shelf bottom water towards the Canada Basin interior has been frequently observed [29] . Therefore, the fluxes of ammonium, DON and silicate were added to the deepest layers just above the shelf bottom in our model so that the simulated nutrient profiles in the Beaufort shelf break were comparable with previous observational results [29] . In addition, to visualize the transport of shelf bottom water, a virtual passive tracer was provided in the deepest layers just above the entire sea bottom. The tracer concentration in the deepest layers was fixed to 1 from May onwards. The tracer value in the water column, except at this bottom layer, was initially zero and could change according to advection and mixing as well as temperature and salinity. Modelled eddy properties We defined ‘eddy grid’, where the absolute value of daily mean relative vorticity exceeded 0.01 f in the southwestern Canada Basin. f is Coriolis parameter at each latitude. The eddy grids were located just above several hundred meters since relative vorticity in the deeper layers was smaller than 0.01 f . The daily mean PON and volume in the eddy grids was horizontally and vertically integrated in the defined southwestern Canada Basin and in the entire water column, respectively. We call these values as ‘Integrated PON of Eddy Grids (IPEG)’ and ‘Integrated Volume of Eddy Grids (IVEG)’, respectively. Besides, the spatially ‘Averaged PON of Eddy Grids’ (APEG) was calculated from daily values of IPEG/IVEG. 0.01 f could be regarded as a lower limit of relative vorticity inside an individual eddy body in the present model experiments. The maximum vorticity was significantly larger at the eddy centres. Even when we chose 0.03 f and 0.05 f , respectively, as the threshold value, there were no significant impacts on our conclusions. How to cite this article: Watanabe, E. et al. Enhanced role of eddies in the Arctic marine biological pump. Nat. Commun. 5:3950 doi: 10.1038/ncomms4950 (2014).